S100A11 is required for efficient plasma membrane repair and survival of invasive cancer cells Cell migration and invasion require increased plasma membrane dynamics and ability to navigate through dense stroma, thereby exposing plasma membrane to tremendous physical stress. Yet, it is largely unknown how metastatic cancer cells acquire an ability to cope with such stress. Here we show that S100A11, a calcium-binding protein upregulated in a variety of metastatic cancers, is essential for efficient plasma membrane repair and survival of highly motile cancer cells. Plasma membrane injury-induced entry of calcium into the cell triggers recruitment of S100A11 and Annexin A2 to the site of injury. We show that S100A11 in a complex with Annexin A2 helps reseal the plasma membrane by facilitating polymerization of cortical F-actin and excision of the damaged part of the plasma membrane. These data reveal plasma membrane repair in general and S100A11 and Annexin A2 in particular as new targets for the therapy of metastatic cancers. Even in the protective environment of a tissue, various mechanical and chemical stresses can damage a cell’s plasma membrane. Accordingly, defect in plasma membrane repair (PMR) is associated with diseases such as muscular dystrophy [1] , diabetes [2] and Chediak–Higashi syndrome [3] . Damaged membrane can be repaired by spontaneous lipid flow across the injured site, outward budding of the damaged membrane and by exocytic fusion of lysosomes and other cytosolic vesicles [4] , [5] , [6] . PMR is triggered by Ca 2+ influx at the injury site, which facilitates cytoskeletal reorganization and membrane fusion events. Cortical cytoskeleton associated with the plasma membrane creates membrane tension, which prevents spontaneous resealing of the membrane [7] . Thus, spatial and temporal remodelling of cortical cytoskeleton at the wound site is essential for efficient PMR [8] . In Xenopus oocytes and Drosophila embryos, membrane injury-induced Ca 2+ influx triggers a decrease in membrane tension through depolymerization of cortical actin cytoskeleton and subsequent formation of a dynamic actin–myosin ring, which contracts and closes the wound in a purse-string manner [9] , [10] . In addition, PMR requires a coordinated interaction between annexin-containing multiprotein complexes and the inner phospholipid surface to seal the rupture [4] . The members of the annexin protein family function as intracellular Ca 2+ sensors. They interact with multiple proteins and distinct anionic phospholipids to promote membrane segregation, vesicle trafficking, vesicle fusion as well as membrane and cytoskeletal organization in a Ca 2+ -dependent manner [11] , [12] . Annexins ANXA1, ANXA6 and ANXA5 regulate PMR by binding the wounded cell membrane and initiating membrane fusion events or forming a protein lattice [13] , [14] , [15] , whereas ANXA2 has been associated with the repair of plasma membrane as well as intracellular vesicle fusion [16] , [17] . Ca 2+ increase also causes members of the S100 family of EF-hand Ca 2+ -binding motif-containing proteins to undergo a conformational change, which exposes a hydrophobic domain of S100 proteins that can interact with the NH 2 -terminal region of some annexins, such as ANXA1 and ANXA2 (ref. 18 ). This interaction is suggested to facilitate close apposition of adjacent phospholipid membranes during a membrane fusion event [19] . However, a role of S100 proteins in cell membrane repair has not been investigated. Increased membrane dynamics and invasion through dense extracellular matrix would expose metastatic cells to membrane stress. Furthermore, malignant transformation is associated with altered membrane stiffness, which together with altered membrane dynamics can lead to stretch-induced membrane pores/ruptures [20] . Yet, the role of PMR in cancer metastasis has not been investigated. It has been reported that annexin-binding protein S100A11 (also known as calgizzarin or metastatic lymph node gene 70 protein) is enriched in pseudopodia of metastatic cancer cells and is essential for the formation of actin-dependent pseudopodial protrusions and tumour cell migration [21] . S100A11 expression is increased in various tumours, and is associated with tumour metastasis as well as poor prognosis in pancreatic, lung and colon cancers [22] , [23] , [24] , [25] , [26] , [27] . We have recently shown that induction of invasive phenotype in MCF7 breast cancer cells by NH 2 terminally truncated 95 kDa form of ErbB2 (p95ErbB2), which mimics the constitutively active cleaved form of ErbB2 oncoprotein commonly found in aggressive breast cancers, is associated with upregulation of S100A11 at the lysosome [28] , [29] . Expression of p95ErbB2 increases invasiveness and mechanical activity of MCF7 (refs 29 , 30 , 31 ). We thus evaluated whether p95ErbB2 increases plasma membrane injury and whether interaction of S100A11 with annexins and lysosome facilitates enhanced PMR. We find that S100A11 depletion does not alter motility, but prevents invasiveness of the MCF7-p95ErbB2 cells by compromising the PMR ability of MCF7- p95ErbB2 cells. S100A11 was not required for injury-triggered lysosome fusion with the plasma membrane. Instead, we found that in vivo , S100A11 forms a complex with Annexin A2 at the site of injury, which facilitates local remodelling of actin cytoskeleton and excision of injured cell membrane. We have thus uncovered an increased need of PMR for invasive cancer cells and show a novel mechanism by which S100A11 helps the invasive cancer cells maintain their plasma membrane integrity. S100A11 protects from invasion associated cell membrane stress We have previously identified S100A11 as a lysosome-associated protein, whose abundance in the lysosomal fraction was increased approximately threefold on p95ErbB2 expression [28] . Notably, p95ErbB2 expression in MCF7 cells increased S100A11 expression by threefold at mRNA and protein levels, the majority of which was localized diffusely in the cytosol ( Fig. 1b ; Supplementary Fig. 1a,b ). This upregulation of S100A11 is mediated by signalling due to p95ErbB2 overexpression, as treating these cells with the MAPK/ERK inhibitor (PD98059) reduced S100A11 protein level in a dose-dependent manner ( Fig. 1c ). 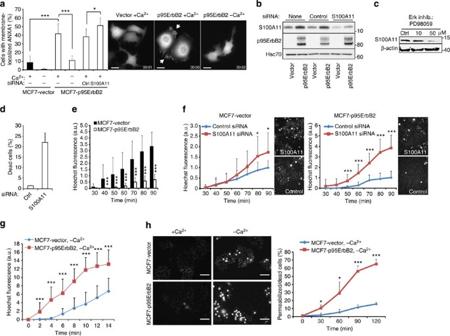Figure 1: S100A11 protects MCF7 cells against p95ErbB2 expression-induced membrane damage. (a) Quantification (left) and representative images (right; scale bar, 20 μm) of ANXA1-GFP-expressing MCF7-vector and -p95ErbB2 cells with membrane-associated ANXA1-GFP after 2 h incubation in a medium with or without Ca2+. When indicated, cells were transfected with control or S100A11-I siRNA 72 h before the experiment. SeeSupplementary Movie 1for the dynamic distribution of ANXA1-GFP in MCF7-p95ErbB2 cells. (b) Representative immunoblot of S100A11 (13 kDa), p95ErbB2 (95 kDa) and Hsc70 (70 kDa; loading control) in lysates of MCF7-vector and -p95ErbB2 cells left untreated or transfected with indicated siRNAs for 72 h. Markers listed represent protein molecular weights in kDa. (c) Immunoblot of S100A11 level in MCF7-p95ErbB2 cells treated for 72 h with Erk inhibitor (inhib.) PD98059. β-actin served as loading control. (d) Cell death assay in MCF7-p95ErbB2 cells 96 h after transfection with control or S100A11-I siRNA as analysed by propidium iodide (PI) exclusion assay and measured by using a fluorescence Celigo imaging cytometer. (e) Permeability of MCF7-vector and -p95ErbB2 cells to Hoechst-33342 under normal growth conditions (30–90 min). Representative images of cells are shown inh(+Ca2+panel). (f) Hoechst-33342 leakage into MCF7-vector and -p95ErbB2 cells treated with indicated siRNAs for 48 h. Fluorescence intensity in each replicate was normalized to that in control siRNA-treated cells 90 min after dye addition. Accompanying images were taken at 90 min. (g) Influx of Hoechst-33342 into MCF7-p95ErbB2 and MCF7-vector cells incubated in Ca2+-free medium as measured every 2 min starting from the time the dye was added to the cells. (h) Representative images of MCF7-vector and -p95ErbB2 cells incubated with Hoechst-33342 in imaging medium±Ca2+for 120 min (left; scale bar, 100 μm) and quantification of permeabilized/dead cells at indicated time points (right). Error bars represent s.d. for a minimum of 20 randomly chosen cells per sample in a representative (n≥3) experiment (aandf–h) or for three independent experiments in triplicate (d). Dead cells with high-intensity staining were excluded from analysis in figuresf–h. All data are representative of a minimum of three independent experiments. The asterisks representP-values based on Student’st-test: *P<0.05; ***P<0.001. Figure 1: S100A11 protects MCF7 cells against p95ErbB2 expression-induced membrane damage. ( a ) Quantification (left) and representative images (right; scale bar, 20 μm) of ANXA1-GFP-expressing MCF7-vector and -p95ErbB2 cells with membrane-associated ANXA1-GFP after 2 h incubation in a medium with or without Ca 2+ . When indicated, cells were transfected with control or S100A11-I siRNA 72 h before the experiment. See Supplementary Movie 1 for the dynamic distribution of ANXA1-GFP in MCF7-p95ErbB2 cells. ( b ) Representative immunoblot of S100A11 (13 kDa), p95ErbB2 (95 kDa) and Hsc70 (70 kDa; loading control) in lysates of MCF7-vector and -p95ErbB2 cells left untreated or transfected with indicated siRNAs for 72 h. Markers listed represent protein molecular weights in kDa. ( c ) Immunoblot of S100A11 level in MCF7-p95ErbB2 cells treated for 72 h with Erk inhibitor (inhib.) PD98059. β-actin served as loading control. ( d ) Cell death assay in MCF7-p95ErbB2 cells 96 h after transfection with control or S100A11-I siRNA as analysed by propidium iodide (PI) exclusion assay and measured by using a fluorescence Celigo imaging cytometer. ( e ) Permeability of MCF7-vector and -p95ErbB2 cells to Hoechst-33342 under normal growth conditions (30–90 min). Representative images of cells are shown in h (+Ca 2+ panel). ( f ) Hoechst-33342 leakage into MCF7-vector and -p95ErbB2 cells treated with indicated siRNAs for 48 h. Fluorescence intensity in each replicate was normalized to that in control siRNA-treated cells 90 min after dye addition. Accompanying images were taken at 90 min. ( g ) Influx of Hoechst-33342 into MCF7-p95ErbB2 and MCF7-vector cells incubated in Ca 2+ -free medium as measured every 2 min starting from the time the dye was added to the cells. ( h ) Representative images of MCF7-vector and -p95ErbB2 cells incubated with Hoechst-33342 in imaging medium±Ca 2+ for 120 min (left; scale bar, 100 μm) and quantification of permeabilized/dead cells at indicated time points (right). Error bars represent s.d. for a minimum of 20 randomly chosen cells per sample in a representative ( n ≥3) experiment ( a and f – h ) or for three independent experiments in triplicate ( d ). Dead cells with high-intensity staining were excluded from analysis in figures f – h . All data are representative of a minimum of three independent experiments. The asterisks represent P -values based on Student’s t -test: * P <0.05; *** P <0.001. Full size image Signalling by the truncated active form of ErbB2 oncoprotein (p95ErbB2) significantly enhances cell motility, membrane ruffling, formation of protrusions and invasiveness of MCF7 breast cancer cells [29] , [32] . This increased activity could lead to increased plasma membrane damage, which may be repaired with help from the S100-binding protein Annexins [4] , [14] , [15] . We thus investigated whether p95ErbB2-induced invasive phenotype of MCF7 cells was associated with increased damage to their plasma membrane. Ca 2+ -dependent recruitment of ANXA1-GFP (green fluorescent protein) to the plasma membrane has been shown to be a marker for plasma membrane damage [33] . We found that compared with 8% of control cells, 40% of MCF7-p95ErbB2 cells displayed extensive plasma membrane association with ANXA1-GFP ( Fig. 1a ; Supplementary Movie 1 ). As changes in phosphoinositide metabolism and increased spontaneous Ca 2+ transients can also increase association of ANXA1-GFP with the cell membrane, we used an independent assay for spontaneous injury and repair of plasma membrane—this involved monitoring the influx of cell membrane-impermeable dye (Hoechst 33342) into live cells. MCF7-p95ErbB2 cells were fivefold more resistant to Hoechst-33342 influx than vector-transfected control cells ( Fig. 1e ). Taken together with the results of ANXA1-GFP reporter, reduced dye leakage indicates that MCF7-p95ErbB2 cells are protected from the effects of increased plasma membrane injury by increased PMR ( Fig. 1a ). We thus tested whether S100A11 overexpression protects MCF7-p95ErbB2 cells from increased membrane damage by depleting the cells of S100A11. S100A11 depletion did not alter the growth ability of the cells, as they showed similar cell cycle profile ( Supplementary Fig. 1g ). However, this increased the cell membrane damage, which was indicated by the increase in number of cells with membrane-recruited ANXA1 ( Fig. 1a ) and an increase in number of dead cells measured by their ability to exclude propidium iodide (PI) ( Fig. 1d ). Further, S100A11 depletion in MCF7-vector and MCF7-p95ErbB2 cells resulted in a greater dye influx in the MCF7-p95ErbB2 (fourfold) as compared with the MCF7-vector cells (1.7-fold) ( Fig. 1f ). While increased Hoechst 33342 labelling requires dye to enter the nucleus, we tested whether any of the dye entry could be due to increased endocytic/pinocytic uptake. For this we tested endocytosis and pinocytosis using lipophilic membrane dye FM1-43 and fluorescence dextran, respectively. We found no significant difference in endocytosis or pinocytosis following S100A11 depletion in HeLa or MCF7-p95ErbB2 cells ( Supplementary Fig. 1c,d ), similarly there was no significant difference between the endocytic rate between MCF7-vector and MCF7-p95ErbB2 cells ( Supplementary Fig. 1e ). In addition, we found that within 2 min of inhibiting PMR (by the removal of Ca 2+ from the medium), there was significantly more influx of Hoechst 33342 in MCF7-p95ErbB2 than in MCF7-vector cells, and this increased dye influx continued linearly thereafter ( Fig. 1g ) such that by 2 h over 65% of MCF7-p95ErbB2 cells died, as compared with only 15% of MCF7-vector cells ( Fig. 1h —plot). Taken together, these data suggest that p95ErbB2-induced transformation results in increased membrane stress and damage, which can be effectively compensated by S100A11- and Ca 2+ -dependent PMR. S100A11 enhances repair of large plasma membrane injuries Next, we investigated whether S100A11 assists in the repair of large plasma membrane injuries. In the first assay, cells were injured by rolling glass beads and then allowed to heal for 5 min. MCF7-p95ErbB2 cells were twice as efficient as MCF7-vector cells at healing from glass bead injury and this efficacy was dependent on the expression of S100A11 in MCF7-p95ErbB2 cells ( Fig. 2a ). In the second assay, we examined the kinetics of PMR by monitoring the entry of membrane-impermeable FM1-43 dye into cells following a laser-induced local injury to the cell membrane. MCF7-p95ErbB2 cells repaired significantly faster than the MCF7-vector cells and the repair efficacy of MCF7-p95ErbB2 cells was compromised by the lack of S100A11 expression ( Fig. 2b ). As an independent test for the role of S100A11 in PMR, we carried out laser injury of HeLa cervical carcinoma cells expressing ANXA1-GFP alone or together with S100A11-RFP (red fluorescent protein). In S100A11-RFP-expressing cells (cell no. 1 in Fig. 2c ; Supplementary Movie 2 ), ANXA1-GFP localized to the site of injury within 10 s of the laser wound and was cleared again within a minute. In S100A11-RFP-negative cells, ANXA1-GFP localized to the proximity of the injury within 10 s but remained localized there even 90 s after the injury, indicating a delay/failure of these cells to heal (cell no. 2 in Fig. 2c ; Supplementary Movie 2 ). These data suggest that S100A11 is not involved in the initial recruitment of ANXA1 to the membrane wound, but instead, enhances the capacity of cells to complete the healing process. The protective ability of ectopic S100A11 in HeLa cells was consistent in a complementary assay where vector- and S100A11-transfected HeLa cells were allowed to repair for 10 min after cell membrane injury by scrape wounding ( Fig. 2d ). Similar to the MCF7 cells, depletion of the endogenous S100A11 in HeLa cells (using three independent short interfering RNAs (siRNAs)) significantly reduced cell viability ( Fig. 2e ). 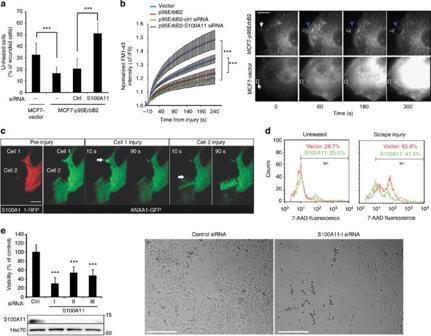Figure 2: S100A11 improves repair of large plasma membrane injuries. (a) Quantification of MCF7-vector and -p95ErbB2 cells that failed to heal (TRITC positive), 5 min following glass bead injury in the presence of FITC-dextran (labels all injured cells). When indicated, cells used were transfected for 72 h with indicated siRNAs. Error bars represent s.d. for a triplicate representative (n=3) experiment with 50–100 randomly chosen wounded cells per condition analysed. (b) Kinetics of cell membrane repair following laser injury. MCF7-vector and -p95ErbB2 cells incubated with FM1-43 dye were injured similarly by laser and the entry of FM1-43 was monitored by measuring FM1-43 intensity following injury (left). Error bars represent s.d. for 10 independent cells per condition. Right panel shows representative images of cells before and after localized laser injury (white arrows). Note that unlike MCF7-vector cell, on injury in MCF7-p95ErbB2 cell the damaged plasma membrane is excised and repaired at a new site marked by blue arrow. (c) Images showing HeLa cells expressing S100A11-RFP and ANXA1-GFP (cell 1) or only ANXA1-GFP (cell 2) before and after localized laser injury (white arrows). Unlike cell 2 that does not overexpress S100A11, cell 1 repairs efficiently as indicated by the rapid clearance of ANXA1-GFP from the injury site; also seeSupplementary Video S2. Scale bar, 20 μm. (d) FACS analysis of 7-AAD entry into uninjured and scrape-injured HeLa cells allowed to repair for 10 min. Values indicate the percentage of cells in the gated area. The results are representative of three independent experiments. (e) Viability of HeLa cells was analysed by MTT reduction assay 96 h after transfection with control or S100A11 siRNAs (top left). Error bars represent s.d. for three independent experiments. Representative immunoblots of S100A11 (13 kDa) and Hsc70 (70 kDa; loading control) in lysates of HeLa cells transfected with indicated siRNAs 72 h before the lysis (bottom left). Representative phase contrast images of cells 96 h after transfection with indicated siRNAs (right). Scale bar, 1 mm. The asterisks representP-values based on Student’st-test: ***P<0.001 when compared as indicated (aandb) or to the control siRNA-treated cells (e). Figure 2: S100A11 improves repair of large plasma membrane injuries. ( a ) Quantification of MCF7-vector and -p95ErbB2 cells that failed to heal (TRITC positive), 5 min following glass bead injury in the presence of FITC-dextran (labels all injured cells). When indicated, cells used were transfected for 72 h with indicated siRNAs. Error bars represent s.d. for a triplicate representative ( n =3) experiment with 50–100 randomly chosen wounded cells per condition analysed. ( b ) Kinetics of cell membrane repair following laser injury. MCF7-vector and -p95ErbB2 cells incubated with FM1-43 dye were injured similarly by laser and the entry of FM1-43 was monitored by measuring FM1-43 intensity following injury (left). Error bars represent s.d. for 10 independent cells per condition. Right panel shows representative images of cells before and after localized laser injury (white arrows). Note that unlike MCF7-vector cell, on injury in MCF7-p95ErbB2 cell the damaged plasma membrane is excised and repaired at a new site marked by blue arrow. ( c ) Images showing HeLa cells expressing S100A11-RFP and ANXA1-GFP (cell 1) or only ANXA1-GFP (cell 2) before and after localized laser injury (white arrows). Unlike cell 2 that does not overexpress S100A11, cell 1 repairs efficiently as indicated by the rapid clearance of ANXA1-GFP from the injury site; also see Supplementary Video S2 . Scale bar, 20 μm. ( d ) FACS analysis of 7-AAD entry into uninjured and scrape-injured HeLa cells allowed to repair for 10 min. Values indicate the percentage of cells in the gated area. The results are representative of three independent experiments. ( e ) Viability of HeLa cells was analysed by MTT reduction assay 96 h after transfection with control or S100A11 siRNAs (top left). Error bars represent s.d. for three independent experiments. Representative immunoblots of S100A11 (13 kDa) and Hsc70 (70 kDa; loading control) in lysates of HeLa cells transfected with indicated siRNAs 72 h before the lysis (bottom left). Representative phase contrast images of cells 96 h after transfection with indicated siRNAs (right). Scale bar, 1 mm. The asterisks represent P -values based on Student’s t -test: *** P <0.001 when compared as indicated ( a and b ) or to the control siRNA-treated cells ( e ). Full size image Taken together, these data support the hypothesis that S100A11 is essential for the efficient repair of externally induced large plasma membrane damage. When imaging the damaged MCF7-p95ErbB2 cells or S100A11-transfected HeLa cells, we frequently observed that the injured part of the cell membrane was excised from the rest of the cell ( Fig. 2b,c , cell no. 1; Supplementary Movie 2 ). Such excision was not observed in MCF7-vector cells or in S100A11-depleted MCF7-p95ErbB2 cells, suggesting that S100A11 may be involved in the excision of the damaged membrane. S100A11 is not required for injury-triggered lysosomal exocytosis Calcium-triggered exocytic fusion of lysosomes with the plasma membrane has been implicated in PMR [5] . As S100A11 can associate with lysosomes [28] , we next examined the putative role of S100A11 in PMR by lysosomal exocytosis. MCF7-p95ErbB2 cells in culture displayed over twofold more lysosome-associated membrane protein 1 (LAMP1) on the cell surface than MCF7-vector cells ( Fig. 3a , white bars). S100A11 depletion caused a twofold increase in cell surface LAMP1 levels in MCF7-vector and MCF7-p95ErbB2 cells, suggesting that S100A11 also has an impact on basal lysosomal exocytosis in MCF7-vector and MCF7-p95ErbB2 cells ( Fig. 3a , black bars). S100A11 depletion also significantly increased basal level of cell surface LAMP1 in HeLa cells ( Fig. 3b ; Supplementary Fig. 1f ). Calcium ionophore treatment of HeLa cells caused a fivefold increase in cell surface LAMP1 and depletion of S100A11 did not alter this fold change ( Fig. 3c ). 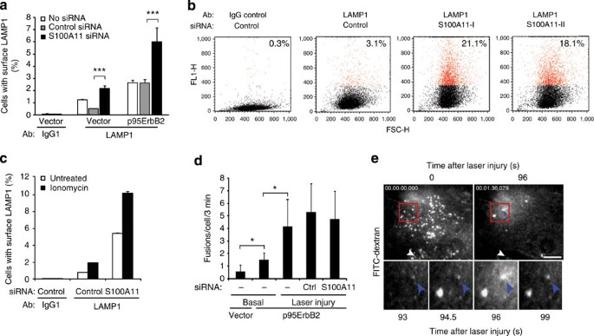Figure 3: S100A11 increases basal, but does not alter injury-dependent lysosomal exocytosis. (a) Quantification of LAMP1 surface staining in MCF7-vector and -p95ErbB2 cells by FACS. When indicated, cells were transfected with appropriate siRNA 72 h before the experiment. Error bars represent s.d. for three independent experiments with 10,000 cells per sample. (b) Representative FACS profiles showing cell surface LAMP1 level (Y-axis) and cell count (X-axis) for HeLa cells transfected with control or S100A11-I siRNAs 72 h prior to the experiment. Red dots indicate M1-gated (cell surface LAMP1 positive) cells. Their percentage is indicated at the top right corner of each plot. SeeFig. 2efor S100A11 knockdown andSupplementary Fig. 1for LAMP1 staining. (c) Quantification of ionomycin-triggered increase in cell surface LAMP1 levels in HeLa cells. Cells were transfected with control or S100A11-I siRNAs 72 h before the experiment and then stained for cell surface LAMP1 before or following treatment with 10 μM ionomycin for 15 min. Error bars represent s.d. for 10,000 cells analysed in a representative experiment. (d) Laser injury-triggered exocytosis by FITC-dextran-labelled lysosomes analysed by TIRF microscopy. Exocytic fusions (flashes of FITC-dextran release) were counted for 3 min in uninjured cells (basal) and for 3 min following laser injury. Error bars represent s.d. for three independent experiments with 5–10 cells per sample analysed. (e) TIRF images of FITC-dextran-labelled lysosomes in a cell before (0 s) and following (96 s) laser injury (top) as well as zoomed in frames from top panel showing a fusing lysosome (bottom). White arrow: site of injury; blue arrow: lysosomal exocytic flash. The asterisks representP-values based on Student’st-test: *P<0.05; ***P<0.001. Figure 3: S100A11 increases basal, but does not alter injury-dependent lysosomal exocytosis. ( a ) Quantification of LAMP1 surface staining in MCF7-vector and -p95ErbB2 cells by FACS. When indicated, cells were transfected with appropriate siRNA 72 h before the experiment. Error bars represent s.d. for three independent experiments with 10,000 cells per sample. ( b ) Representative FACS profiles showing cell surface LAMP1 level (Y-axis) and cell count (X-axis) for HeLa cells transfected with control or S100A11-I siRNAs 72 h prior to the experiment. Red dots indicate M1-gated (cell surface LAMP1 positive) cells. Their percentage is indicated at the top right corner of each plot. See Fig. 2e for S100A11 knockdown and Supplementary Fig. 1 for LAMP1 staining. ( c ) Quantification of ionomycin-triggered increase in cell surface LAMP1 levels in HeLa cells. Cells were transfected with control or S100A11-I siRNAs 72 h before the experiment and then stained for cell surface LAMP1 before or following treatment with 10 μM ionomycin for 15 min. Error bars represent s.d. for 10,000 cells analysed in a representative experiment. ( d ) Laser injury-triggered exocytosis by FITC-dextran-labelled lysosomes analysed by TIRF microscopy. Exocytic fusions (flashes of FITC-dextran release) were counted for 3 min in uninjured cells (basal) and for 3 min following laser injury. Error bars represent s.d. for three independent experiments with 5–10 cells per sample analysed. ( e ) TIRF images of FITC-dextran-labelled lysosomes in a cell before (0 s) and following (96 s) laser injury (top) as well as zoomed in frames from top panel showing a fusing lysosome (bottom). White arrow: site of injury; blue arrow: lysosomal exocytic flash. The asterisks represent P -values based on Student’s t -test: * P <0.05; *** P <0.001. Full size image In another approach, we directly monitored the exocytic activity of FITC-dextran-labelled lysosomes (bursts of dextran release to the extracellular space) in untreated cells and in response to laser injury by total internal reflection microscopy [34] , [35] . In agreement with increased cell surface LAMP1 staining ( Fig. 3a ), the basal exocytic activity was doubled by the expression of p95ErbB2 ( Fig. 3d ). Laser injury triggered an S100A11-independent fourfold increase in the number of lysosome exocytosis events, and these fusions spread throughout the cell and not specifically around the injury site ( Fig. 3d,e ). Thus, S100A11 is not needed for lysosomal exocytosis and the increased basal lysosomal exocytosis in S100A11-depleted cells may reflect an increased influx of Ca 2+ as a consequence of defective PMR. Ca 2+ -triggers S100A11-ANXA2 interaction at the site of repair To gain insight into the mechanism by which S100A11 regulates PMR, we monitored localization of S100A11 and potential binding partners ANAX1 and ANXA2. Within 30 s of the laser injury of MCF7-p95ErbB2 cells expressing GFP- and RFP-tagged pair of these proteins, ANXA1 and S100A11 began to accumulate around the site of injury, reaching a maximum accumulation by 150 s ( Fig. 4a ; Supplementary Fig. 2a,b ; Supplementary Movie 3 ). As the repair proceeded, ANXA1 localized to the injured membrane that was eventually excised, whereas S100A11 was localized to the repairing cell membrane ( Fig. 4a ; Supplementary Fig. 2a,b ; Supplementary Movie 3 ). After repair and excision of the injured membrane, S100A11 diffused back into the cytosol within the next 100 s, while ANXA1 remained at the injured and excised membrane ( Supplementary Fig. 2a ; Supplementary Movie 3 ). In the absence of Ca 2+ , ANXA1 and S100A11 leaked out of the damaged cell, failing to accumulate at the site of injury ( Supplementary Fig. 2c ). 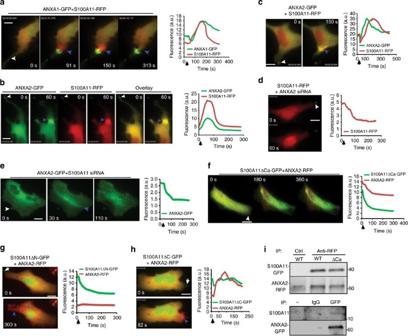Figure 4: S100A11 forms a complex with ANXA2 and co-operate at the site of PMR. (a) Images and plots showing the kinetics and localization of fluorescently tagged S100A11 and ANXA1 in response to laser injury (white arrows: site of injury) in MCF7-p95ErbB2. (b,c) Images and plots showing the kinetics of accumulation of S100A11-RFP and ANXA2-GFP following laser injury in (b) MCF7-p95ErbB2 cells and (c) HeLa cells. Site of repair is indicated by blue arrows. (d) S100A11-RFP and (e) ANXA2-GFP accumulation at the site of injury (white arrowhead) monitored in HeLa cells 48 h after silencing the expression of ANXA2 and S100A11, respectively. (f–h) HeLa cells expressing ANXA2-RFP and different S100A11-mutant proteins including (f) S100A11ΔCa-GFP, (g) S100A11ΔN-GFP or (h) S100A11ΔC-GFP were injured by laser (injury site: white arrow) and imaged by time-lapse microscopy. Results are representative of at least five experiments. Wherever indicated, blue arrowheads mark the site of repair. Scale bar, 20 μm. (i) Representative co-immunoprecipitation using RFP or control antibodies from lysates of HeLa cells expressing ANXA2-RFP and S100A11-GFP and exposed to scrape injury (WT/mutant). The panel below shows western blot analysis of endogenous S100A11 co-IP using GFP antibody to pull-down ANXA2-GFP from lysate of MCF7-p95ErbB2 cells expressing only ANXA2-GFP. This lysate was split into three parts and incubated with no antibody (−), mouse IgG2 (IgG) or anti-GFP monoclonal antibody (GFP). Following IP, western blot analysis was carried out using S100A11 antibody. Figure 4: S100A11 forms a complex with ANXA2 and co-operate at the site of PMR. ( a ) Images and plots showing the kinetics and localization of fluorescently tagged S100A11 and ANXA1 in response to laser injury (white arrows: site of injury) in MCF7-p95ErbB2. ( b , c ) Images and plots showing the kinetics of accumulation of S100A11-RFP and ANXA2-GFP following laser injury in ( b ) MCF7-p95ErbB2 cells and ( c ) HeLa cells. Site of repair is indicated by blue arrows. ( d ) S100A11-RFP and ( e ) ANXA2-GFP accumulation at the site of injury (white arrowhead) monitored in HeLa cells 48 h after silencing the expression of ANXA2 and S100A11, respectively. ( f – h ) HeLa cells expressing ANXA2-RFP and different S100A11-mutant proteins including ( f ) S100A11ΔCa-GFP, ( g ) S100A11ΔN-GFP or ( h ) S100A11ΔC-GFP were injured by laser (injury site: white arrow) and imaged by time-lapse microscopy. Results are representative of at least five experiments. Wherever indicated, blue arrowheads mark the site of repair. Scale bar, 20 μm. ( i ) Representative co-immunoprecipitation using RFP or control antibodies from lysates of HeLa cells expressing ANXA2-RFP and S100A11-GFP and exposed to scrape injury (WT/mutant). The panel below shows western blot analysis of endogenous S100A11 co-IP using GFP antibody to pull-down ANXA2-GFP from lysate of MCF7-p95ErbB2 cells expressing only ANXA2-GFP. This lysate was split into three parts and incubated with no antibody (−), mouse IgG2 (IgG) or anti-GFP monoclonal antibody (GFP). Following IP, western blot analysis was carried out using S100A11 antibody. Full size image On injury, simultaneously with S100A11, ANXA2 also accumulated at the injury site ( Fig. 4b,c ). However, unlike ANXA1, following injury-triggered accumulation, ANXA2 was cleared simultaneously with S100A11 at the repairing membrane in injured MCF7-p95ErbB2 ( Fig. 4b —plot) and HeLa cells ( Fig. 4c —plot; Supplementary Movie 4 ). Depletion of ANXA2 in HeLa cells by using ANXA2-siRNA ( Supplementary Fig. 2d ) prevented the accumulation of S100A11 ( Fig. 4d ), and vice versa depletion of S100A11 ( Fig. 2e ) prevented the accumulation of ANXA2 at the repair site ( Fig. 4e ). These results together with the reported ability of ANXA2 and S100A11 to interact with each other in vitro [36] suggested that ANXA2 and S100A11 are recruited to the site of repair as a complex. Thus, it is interesting to note that akin to S100A11, the expression of ANXA2 was significantly upregulated by p95ErbB2 in MCF7 cells ( Supplementary Fig. 2d ). To investigate the molecular details of S100A11 and ANXA2 interaction during PMR, we used three S100A11 mutants; S100A11ΔCa lacking the Ca 2+ -binding domain essential for Ca 2+ -induced conformational changes and S100A11–ANXA2 interaction [37] , S100A11ΔN lacking 23 amino acids at the NH 2 terminus essential for S100A11–ANXA2 interaction [36] and S100A11ΔC lacking 19 amino acids at the C terminus, suggested to interact with actin [37] . We transfected HeLa cells with these S100A11 mutants tagged with GFP and monitored their injury-triggered trafficking and effects on the trafficking of RFP-tagged ANXA2 as well as wild-type (WT) S100A11. Contrary to the WT S100A11 ( Fig. 4a–c ), all three mutants failed to translocate to the injury site ( Fig. 4f–h ). In a dominant negative manner, S100A11ΔCa ( Fig. 4f ; Supplementary Fig. 2e ) and S100A11ΔN ( Fig. 4g ), but not S100A11ΔC ( Fig. 4h ), prevented the recruitment of ANXA2 ( Fig. 4f–h ) and WT S100A11 ( Supplementary Fig. 2e ) to the damaged membrane. To examine interaction between ANXA2 and S100A11 proteins, we carried out co-immunoprecipitation (co-IP) experiment using RFP antibody in HeLa cells co-expressing ANXA2-RFP and WT or mutant S100A11-GFP. Following scrape injury, anti-RFP antibody was able to co-IP ANXA2-RFP with WT and ΔCa S100A11 mutant, indicating the ability of ANXA2 to form a complex with these S100A11 proteins ( Fig. 4i , upper panel). Further, IP with GFP antibody in MCF7-p95ErbB2 cells expressing ANXA2-GFP resulted in co-IP of endogenous S100A11 protein from these cells ( Fig. 4i , lower panel). A characteristic feature of the S100 family of calcium-binding proteins is that they form non-covalent homodimers [18] . Thus, the dominant negative effect of S100A11ΔCa and S100A11ΔN further suggests that S100A11 and ANXA2 are recruited to the injury site as a complex. S100A11–ANXA2 complex augments PMR by altering local actin dynamics In view of the ability of S100A11 to bind F-actin in a Ca 2+ -dependent manner [38] , [39] and of ANXA2 to regulate the formation and growth of F-actin bundles [12] , [40] together with the need of F-actin assembly to control PMR in other organisms [9] , [41] , we tested whether S100A11 and ANXA2 regulate PMR by regulating actin dynamics in human cells. Our previous in vitro studies have identified that GST-tagged S100A11 protein interacts with F-actin (not G-actin) in a dose-dependent manner [38] . We carried out co-IP experiment by expressing S100A11-tGFP in HeLa cells and confirmed in vivo interaction of S100A11 with β-actin ( Fig. 5a ). In uninjured cells, S100A11 and β-actin distributed uniformly throughout the cells, but glass bead-induced plasma membrane injury caused co-accumulation of β-actin and S100A11 at the damaged membranes ( Fig. 5b ). Immediately following laser-induced plasma membrane injury and before the accumulation of S100A11, the level of β-actin at the site of injury decreased ( Fig. 5c ). This was followed by the accumulation of S100A11 and the subsequent buildup of β-actin ( Fig. 5c ; Supplementary Fig. 3a ; Supplementary Movie 5 ). On completion of PMR, both proteins returned back to their pre-injury distribution at the repair site. 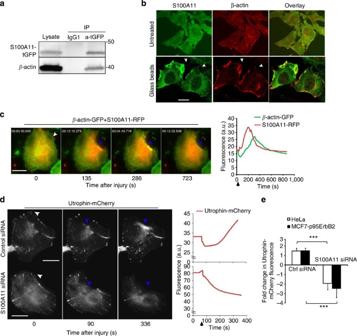Figure 5: S100A11 is required for F-actin buildup at the site of PMR. (a) Representative immunoblots of lysates of HeLa cells expressing S100A11-tGFP before or after immunoprecipitation using anti-tGFP or control IgG1 antibody and probed with S100A11 as well as β-actin antibodies. (b) Images of HeLa cells stained for endogenous S100A11 and β-actin after glass bead injury. Colocalization of the two proteins at the damaged membrane is indicated by arrowheads. (c) Images (left) of S100A11-RFP and β-actin-GFP recruitment to the repair site (blue arrowheads) in a HeLa cell following a local laser injury (white arrow). Corresponding plot (right) shows change in fluorescence intensity of these two proteins at the site of repair (blue arrowheads).Supplementary Figure S3Ashows the images of individual channels andSupplementary Video S5shows the dynamics of this process. (d) HeLa cells expressing endogenous S100A11 or knocked down for S100A11 were transfected with Utrophin-mCherry and its accumulation at the site of repair (blue arrow) was imaged (left panel andSupplementary Video S6) and quantified (right) at the repair site in live cells. (e) Average fold change in Utrophin-mCherry fluorescence around the repair site in HeLa and MCF7-p95ErbB2 cells was quantified in each case for 5–7 cells, black arrows mark the time of injury. Also seeSupplementary Fig. S3B. ***P<0.001. Scale bar, 20 μm. Figure 5: S100A11 is required for F-actin buildup at the site of PMR. ( a ) Representative immunoblots of lysates of HeLa cells expressing S100A11-tGFP before or after immunoprecipitation using anti-tGFP or control IgG1 antibody and probed with S100A11 as well as β-actin antibodies. ( b ) Images of HeLa cells stained for endogenous S100A11 and β-actin after glass bead injury. Colocalization of the two proteins at the damaged membrane is indicated by arrowheads. ( c ) Images (left) of S100A11-RFP and β-actin-GFP recruitment to the repair site (blue arrowheads) in a HeLa cell following a local laser injury (white arrow). Corresponding plot (right) shows change in fluorescence intensity of these two proteins at the site of repair (blue arrowheads). Supplementary Figure S3A shows the images of individual channels and Supplementary Video S5 shows the dynamics of this process. ( d ) HeLa cells expressing endogenous S100A11 or knocked down for S100A11 were transfected with Utrophin-mCherry and its accumulation at the site of repair (blue arrow) was imaged (left panel and Supplementary Video S6 ) and quantified (right) at the repair site in live cells. ( e ) Average fold change in Utrophin-mCherry fluorescence around the repair site in HeLa and MCF7-p95ErbB2 cells was quantified in each case for 5–7 cells, black arrows mark the time of injury. Also see Supplementary Fig. S3B . *** P <0.001. Scale bar, 20 μm. Full size image To test whether S100A11–ANXA2 complex regulates F-actin dynamics at the repair site, we probed F-actin with Utrophin-mCherry [42] . In HeLa cells, in the presence of endogenous S100A11, ANXA1 was rapidly recruited to the injured part of the plasma membrane (not shown) followed by localized F-actin buildup at the site of repair ( Fig. 5d ; Supplementary Movie 6 ). Depletion of S100A11 prevented F-actin accumulation completely. Besides, the level of F-actin around the injured membrane declined rapidly and the cell failed to repair the membrane ( Fig. 5d,e ). A similar S100A11-dependent increase in the level of Utrophin-mCherry near the injured membrane was observed in MCF7-p95ErbB2 cells ( Fig. 5e ; Supplementary Fig. 3b ). Thus, S100A11–ANXA2 complex may regulate membrane repair by facilitating cortical actin polymerization beneath the injury site, thereby assisting the closure of the wound. Time-lapse imaging of the repair process in laser-injured cells revealed that S100A11 was recruited to the injury site in waves, each wave of S100A11 correlating with a subsequent increase in F-actin buildup ( Fig. 6a ; Supplementary Movie 7 ). This process was absent in cells expressing the dominant negative S100A11ΔCa mutant ( Fig. 6b ), which inhibited S100A11–ANXA2 complex recruitment to the injured membrane ( Fig. 4f ; Supplementary Fig. 2e ). Supporting the importance of actin dynamics in the repair process, inhibition of F-actin remodelling by either cytochalasin D (actin polymerization inhibitor) or jasplakinolide (actin depolymerization inhibitor) also significantly impaired PMR after local laser injury ( Fig. 6c ). This occurred to the extent that many drug-treated cells were severely damaged as illustrated by the accumulation of ANXA1-GFP to the large parts of the membrane ( Fig. 6d ). Altering F-actin dynamics by treatment with either cytochalasin D or jasplakinolide did not affect the ability of S100A11 ( Fig. 6e ) to accumulate at the site of injury. These proteins remained, however, at the site of injury 4–5 times longer than in untreated control cells ( Fig. 6e,f ). These findings suggest that accumulation of S100A11 and ANXA2 at the injured membrane is independent of F-actin dynamics, but normal F-actin assembly and disassembly are required for effective PMR and clearance of S100A11–ANXA2 complex from the membrane. 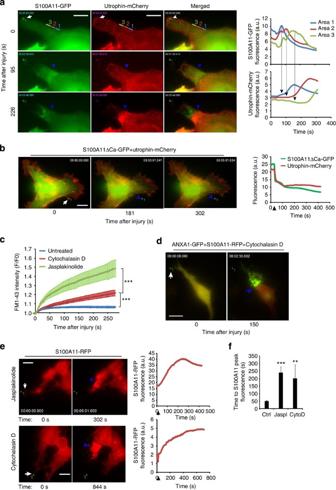Figure 6: S100A11–ANXA2 complex augments PMR by altering local actin dynamics. (a) Images (left) of HeLa cells showing waves of recruitment of S100A11-GFP and F-actin (marked by Utrophin-mCherry) at the site of repair (areas 1–3) following laser injury (white arrow). Corresponding fluorescence intensity plots (right) reflect the presence of the indicated proteins in the coloured areas marked 1, 2 and 3 before and after the injury.Supplementary Movie 7shows the entire kinetics. (b) Representative images (left) of S100A11ΔCa-GFP and Utrophin-mCherry recruitment to the repair site (blue arrowheads) in a HeLa cell following a local laser injury (white arrow). Corresponding plot (right) shows fluorescence intensity of the indicated proteins at the repair site. (c) Kinetics of repair following focal laser injury of HeLa cells pretreated with 20 μM cytochalasin D (cyto D) for >30 min or with 0.5 μM jasplakinolide (Jaspl) for >30 min, as measured by FM1-43 dye-uptake approach described inFig. 2b. Each curve is an average of 10 cells. ***P<10−3(at 275 s) based on Student’st-test. (d) Image showing the extent of cell membrane injury as marked by ANXA1-GFP accumulation in a HeLa cell pretreated with cytochalasin D for 30 min before laser injury. (e) Representative images (left) of HeLa cells expressing S100A11-RFP and treated with jasplakinolide for 120 min or with Cytochalasin D for 80 min before laser injury. Corresponding plots show the kinetics of S100A11-RFP recruitment at the site of repair (blue arrowhead). (f) Time for peak S100A11 accumulation at the repair site following laser injury of HeLa cells untreated (Ctrl) or treated as ine. Error bars represent s.d. for >5 independent experiments. The asterisks representP-values based on Student’st-test: **P<0.01; ***P<0.001 when compared with untreated control cells. Scale bar, 20 μm. Figure 6: S100A11–ANXA2 complex augments PMR by altering local actin dynamics. ( a ) Images (left) of HeLa cells showing waves of recruitment of S100A11-GFP and F-actin (marked by Utrophin-mCherry) at the site of repair (areas 1–3) following laser injury (white arrow). Corresponding fluorescence intensity plots (right) reflect the presence of the indicated proteins in the coloured areas marked 1, 2 and 3 before and after the injury. Supplementary Movie 7 shows the entire kinetics. ( b ) Representative images (left) of S100A11ΔCa-GFP and Utrophin-mCherry recruitment to the repair site (blue arrowheads) in a HeLa cell following a local laser injury (white arrow). Corresponding plot (right) shows fluorescence intensity of the indicated proteins at the repair site. ( c ) Kinetics of repair following focal laser injury of HeLa cells pretreated with 20 μM cytochalasin D (cyto D) for >30 min or with 0.5 μM jasplakinolide (Jaspl) for >30 min, as measured by FM1-43 dye-uptake approach described in Fig. 2b . Each curve is an average of 10 cells. *** P <10 −3 (at 275 s) based on Student’s t -test. ( d ) Image showing the extent of cell membrane injury as marked by ANXA1-GFP accumulation in a HeLa cell pretreated with cytochalasin D for 30 min before laser injury. ( e ) Representative images (left) of HeLa cells expressing S100A11-RFP and treated with jasplakinolide for 120 min or with Cytochalasin D for 80 min before laser injury. Corresponding plots show the kinetics of S100A11-RFP recruitment at the site of repair (blue arrowhead). ( f ) Time for peak S100A11 accumulation at the repair site following laser injury of HeLa cells untreated (Ctrl) or treated as in e . Error bars represent s.d. for >5 independent experiments. The asterisks represent P -values based on Student’s t -test: ** P <0.01; *** P <0.001 when compared with untreated control cells. Scale bar, 20 μm. Full size image S100A11 is required for tumour cell invasiveness As we have reported before [29] , p95ErbB2 expression also provided MCF7 cells with a capacity to invade into 3-dimensional (3D) matrigel matrix, a process that exposes cell membranes to an even higher degree of physical stress. In view of our above findings that invasive phenotype triggered by p95ErbB2 overexpression is associated with increased need for PMR by S100A11 and ANXA2, we investigated whether blocking S100A11-dependent PMR machinery would compromise the invasive phenotype. Unlike MCF7-p95ErbB2 cells transfected with control siRNA that migrated out of the matrigel matrix, S100A11-depleted MCF7-p95ErbB2 cells resembled the MCF7-vector cells that formed non-invading compact spheroids ( Fig. 7a ). In view of the involvement of S100A11 in metastatic cell migration [21] , we examined whether reduced invasiveness of S100A11-depleted MCF7-p95ErbB2 cells reflects loss in cell mobility. We monitored motility of MCF7-p95ErB2 cells treated for 72 h with S100A11-specific or control siRNA and found no difference in mean cellular velocity of these cells ( Fig. 7b ). In addition, unlike improved PMR of HeLa cells overexpressing S100A11 ( Fig. 2c ), overexpression of S100A11 did not enhance the motility of HeLa cells to migrate into and close a gap in a cell monolayer created by scratching of the cell monolayer ( Fig. 7c ). These findings suggest that despite normal cellular motility, poor PMR can restrict the invasive ability of MCF7-p95ErbB2 cells in 3D matrigel matrix. 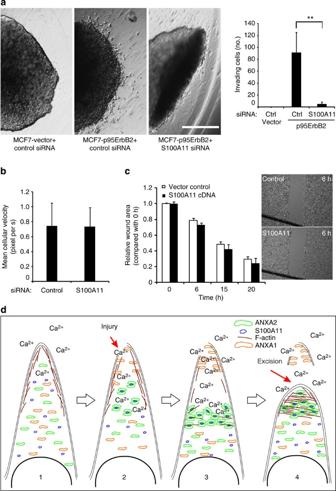Figure 7: S100A11 is required for the invasiveness of MCF7-p95ErbB2 cells. (a) MCF7-vector and -p95ErbB2 cells expressing indicated siRNAs were grown in hanging drops overnight. Multicellular spheroids were subsequently grown for 2 days as spheroid cultures in a thin matrix of Matrigel. The spheroids were imaged with transmitted light to monitor the invasive growth of cells (left). Scale bar, 1 mm. Plot (right) shows the quantification of invading cells from spheroids. Error bars represent s.d. for four independent spheroids. On the basis of Student’st-test, **P<0.01. (b) Sparsely seeded MCF7-p95ErbB2 cells treated with the indicated siRNAs for 72 h were tracked for 6 h. Mean cellular velocity was quantified for 30 cells in each condition; error bars represent s.d. This data is representative of three independent experiments. (c) Analysis of the directional motility of HeLa cells expressing S100A11 or empty vector (control). Confluent monolayer of HeLa cells was disrupted to generate a gap to facilitate directional migration of cells. The edge of the gap in the monolayer (monolayer wound area) was quantified and wound distance calculated relative to 0 h. Inset shows representative images of monolayers after 6 h of cell migration. Error bars represent s.d. for three independent experiments. Scale bar, 1 mm. (d) Proposed model for cell membrane repair mediated by S100A11–ANXA2 complex. In uninjured cell: (1) cortical actin maintains high tension of the plasma membrane and with the low cytosolic Ca2+ANXA1, ANXA2 and S100A11 are distributed uniformly throughout the cytosol. (2) Local injury. (3) Causes increase in cytosolic Ca2+, resulting in accumulation of ANXA1 at the injury site, depolymerization of F-actin at this site and accumulation of S100A11–ANXA2 complex proximal to the injury site. (4) Actin depolymerization reduces the local membrane tension, causing the wounded membrane surrounding the site of injury to collapse onto each other and separate from the damaged part of the cell membrane. The S100A11–ANXA2 complex initiates F-actin polymerization at this site, which aids in the fusion of the injured membrane at the repair site and helps re-establish the membrane tension to support the newly formed cell membrane and facilitate complete wound closure. Figure 7: S100A11 is required for the invasiveness of MCF7-p95ErbB2 cells. ( a ) MCF7-vector and -p95ErbB2 cells expressing indicated siRNAs were grown in hanging drops overnight. Multicellular spheroids were subsequently grown for 2 days as spheroid cultures in a thin matrix of Matrigel. The spheroids were imaged with transmitted light to monitor the invasive growth of cells (left). Scale bar, 1 mm. Plot (right) shows the quantification of invading cells from spheroids. Error bars represent s.d. for four independent spheroids. On the basis of Student’s t -test, ** P <0.01. ( b ) Sparsely seeded MCF7-p95ErbB2 cells treated with the indicated siRNAs for 72 h were tracked for 6 h. Mean cellular velocity was quantified for 30 cells in each condition; error bars represent s.d. This data is representative of three independent experiments. ( c ) Analysis of the directional motility of HeLa cells expressing S100A11 or empty vector (control). Confluent monolayer of HeLa cells was disrupted to generate a gap to facilitate directional migration of cells. The edge of the gap in the monolayer (monolayer wound area) was quantified and wound distance calculated relative to 0 h. Inset shows representative images of monolayers after 6 h of cell migration. Error bars represent s.d. for three independent experiments. Scale bar, 1 mm. ( d ) Proposed model for cell membrane repair mediated by S100A11–ANXA2 complex. In uninjured cell: (1) cortical actin maintains high tension of the plasma membrane and with the low cytosolic Ca 2+ ANXA1, ANXA2 and S100A11 are distributed uniformly throughout the cytosol. (2) Local injury. (3) Causes increase in cytosolic Ca 2+ , resulting in accumulation of ANXA1 at the injury site, depolymerization of F-actin at this site and accumulation of S100A11–ANXA2 complex proximal to the injury site. (4) Actin depolymerization reduces the local membrane tension, causing the wounded membrane surrounding the site of injury to collapse onto each other and separate from the damaged part of the cell membrane. The S100A11–ANXA2 complex initiates F-actin polymerization at this site, which aids in the fusion of the injured membrane at the repair site and helps re-establish the membrane tension to support the newly formed cell membrane and facilitate complete wound closure. Full size image Our results demonstrate that MCF7 breast cancer cells made metastatic by ectopic expression of p95ErbB2 oncoprotein require enhanced PMR through increased expression of S100A11 and ANXA2 proteins. As a result of enhanced PMR, these cells are more efficient than the non-invasive MCF7 cells at maintaining plasma membrane integrity following various stresses and injuries due to their invasive nature. Accordingly, loss of S100A11–ANXA2 complex reduces their viability and compromises their invasive ability. These observations indicate that repairing injured cell membranes is critical for survival and metastasis, and thus explain the need for high S100A11 levels in metastatic cells of various origins [25] , [26] , [27] . ANXA1, a binding partner of S100A11, is recruited to the injured cell membrane in a Ca 2+ -dependent manner, presumably to initiate repair response [14] . However, the recruitment of ANXA1 at the site of injury is independent of S100A11 binding, as it persists in cells lacking S100A11. Moreover, ANXA1 accumulates at the damaged part of the cell that is eventually excised, while S100A11 is recruited to the site where new cortical actin builds up and helps with the excision of the damaged cell membrane. Our data offer the first clear demonstration of such an excision process and provide the underlying mechanism regulating this process. Unlike ANXA1, we find that ANXA2 colocalizes with S100A11 at the injury site and their presence at the repair site is mutually dependent. This is in line with the fivefold tighter Ca 2+ -dependent in vitro interaction of S100A11 with ANXA2 as compared with ANXA1 (ref. 36 ). Mutation in S100A11 that prevents its Ca 2+ binding or deletions of either NH 2 or C terminus inhibits the ability of S100A11 to localize to the site of injury and inhibits PMR. This is consistent with the requirements of S100A11 NH 2 -terminal amino acids and Ca 2+ -induced conformational change for S100A11–ANXA2 interaction [36] , [38] . Our data demonstrates that the key function of S100A11–ANXA2 complex in PMR is to aid in remodelling of actin cytoskeleton at the site of injury to facilitate excision of the damaged cell membrane. This function of S100A11–ANXA2 complex is in agreement with work showing individual interactions of S100A11 and ANXA2 proteins with the actin cytoskeleton [12] , [38] . The participation of actin in the cell membrane repair process has been shown to be important in Xenopus oocytes and Drosophila embryo [9] , [10] . Thus, actin appears to be the evolutionarily conserved facilitator of cell membrane repair. While the involvement of S100 in PMR has not been examined in these model systems, annexins have been shown to regulate PMR in zebrafish [43] . It is not known whether annexin-mediated PMR in zebrafish involves modulation of actin cytoskeleton. Here we show that S100A11–ANXA2 complex interacts with β-actin and that it is required for the proper remodelling of actin to facilitate wound closure in mammalian cells. The important role of actin dynamics in this process is further supported by inhibition of PMR by drugs that block actin polymerization or depolymerization [41] . We propose that this is due to the role of membrane-associated cortical actin cytoskeleton in maintaining cell membrane stability. While cortical F-actin is necessary to support the cell membrane, it also creates tension that would inhibit passive resealing after injury [7] . Thus, depolymerizing cortical actin after injury would not only keep the tension from further damaging the injured cell membrane, but will also facilitate membrane fusion to enhance the repair of the wounded membrane [44] . Localized wounding of 3T3 fibroblasts has been shown to significantly reduce membrane tension in a Ca 2+ -dependent manner [7] . This could be due to the cortical actin depolymerization triggered by calcium-induced activation of F-actin-severing proteins such as gelsolin [45] . Loss of tension and clearance of cortical actin together with increased cell membrane access for vesicles can contribute to the repair of the wounded membrane [44] . On the basis of our observations, we have proposed a model that depicts the various steps during PMR ( Fig. 7d ). In resting cell, ANXA1, ANXA2 and S100A11 are predominantly cytosolic and there is a layer of cortical actin under the cell membrane. Following cell membrane injury, the cortical F-actin consistently decreases around the injury site concomitant with the recruitment of ANXA1 at the injured cell membrane. We propose that Ca 2+ -triggered local loss of F-actin by actin-severing proteins reduces membrane tension and brings together the wounded edges of the cell membrane ( Fig. 7d ). This is followed by Ca 2+ -dependent accumulation of S100A11–ANXA2 complex near the injury site. As S100A11 and ANXA2 bind F-actin and decrease the depolymerization rate of preformed actin filaments [12] , [38] , the S100A11–ANXA2 complex restricts F-actin depolymerization, preserving and allowing new buildup of F-actin around the injury site. ANXA2 is also capable of Ca 2+ -dependent binding to phospholipids, which enables aggregation of endosomes and other vesicles [46] . At these membranes, the S100A11–ANXA2 complex helps nucleate polymerization of cortical F-actin by enabling buildup of cortical F-actin [40] . The buildup of the cortical F-actin together with presence of vesicular endomembrane and the wounded edges of the plasma membrane, all participate in the fusion of the wounded cell membrane at the repair site marked by the S100A11–ANXA2 complex and the excision of the damaged part of the cell membrane marked by ANXA1. The buildup of cortical actin we observe here is analogous to F-actin drawstring formation during healing of injured Xenopus oocyte cell membrane [9] . Thus, we propose that the F-actin buildup allows pulling the wounded membrane edges together during excision to facilitate repair. Recently, it has been shown that Ca 2+ -regulated cyclic assembly and disassembly of F-actin at the cell membrane regulates vesicle fusion [47] . Thus, the vesicle aggregation and F-actin assembly mediated by the S100A11–ANXA2 complex may help with PMR by facilitating vesicle fusion and cortical actin buildup. Lysosomes are among the vesicles whose Ca 2+ -triggered fusion has been linked to PMR [5] . Accordingly, Ca 2+ influx caused by injury or ionomycin resulted in an increase in lysosome exocytosis. However, extent of lysosomal exocytosis is unaltered by S100A11 expression. S100A11 depletion does result in increased basal lysosomal exocytosis, but this is likely due to the poor repair following spontaneous plasma membrane damage in S100A11-depleted cells. While S100A11–ANXA2 complex does not regulate lysosome exocytosis in response to injury, it remains plausible that this complex regulates the fusion of other vesicles involved in PMR [35] . S100A11 localized to nucleus has been shown to inhibit keratinocyte growth liberating Sp1/3 from nucleolin to activate the negative cell cycle regulator p21 CIP1/WAF1 , whereas secreted S100A11 can activate cell growth [37] , [48] . To this end, our results identify that maintaining plasma membrane integrity is a key intracellular function of S100A11 in the metastatic cells. This functional duality of S100A11 may benefit by linking large membrane injury to G1 cell cycle arrest, thus keeping injured cells from entering cell division until they have successfully recovered. Our finding of a role of S100A11 in regulating cell membrane and associated cytoskeleton adds to a recent study of six metastatic cancer cell lines, which reported significant reduction in pseudopod formation and invasion after S100A11 knockdown [21] . It is interesting to note that all of these processes are dependent on the function of the actomyosin complex, defects in which we have found to be responsible for the poor PMR in these cells. In summary, our study demonstrates that metastatic cancer cells have elevated rate of cell injury and that they rely on the S100A11–ANXA2 complex to enable cell membrane repair. The repair response proceeds by excision of the damaged part of the cell membrane. Our findings suggest that the S100A11–ANXA2 complex, injury-triggered actin remodelling and other steps in the PMR response are novel and viable targets for controlling tumour cell metastasis. Cell culture and treatments MCF7 and HeLa cells originate from human breast carcinoma and cervix carcinoma, respectively, and were obtained from ATCC. MCF7-p95ErbB2 and MCF7-pTRE cell lines are single cell clones of MCF7 expressing the tetracycline transactivator transfected with pTRE-p95ErbB2 and pTRE, respectively [32] . To induce p95ErbB2 expression, tetracycline (1 μg ml −1 ) was removed and cells were washed five times in PBS before plating. siRNAs and plasmid constructs For all siRNAs knockdown, 20 nM siRNA was used. Sequence of the siRNAs used is listed in Supplementary Table 1 . Control siRNA: AllStar Negative Control siRNA (QIAGEN). Plasmids: Human S100A11-turboGFP/S100A11-turboRFP with C-terminal GFP tag were purchased from OriGene Technologies. ANXA1-GFP was kindly obtained from ref. 49 , ANXA2-GFP/RFP from Deora et al. [50] and Utrophin-mCherry from William Bement [42] . The S100A11 deletion mutants were similar to before [37] and constructed as GFP fusions in the manner described below. To eliminate Ca 2+ -binding capacity, by site-directed mutagenesis amino acids 38E in the loop 1 and 72D, 76D and 79E in the loop 2 were changed to S (S100A11ΔCa). For S100A11ΔN, human S100A11 cDNA lacking 23 amino acids from the N terminus and for S100A11ΔC, human S100A11 cDNA lacking 19 amino acids from C terminus were obtained by PCR and the DNA sequence confirmed. The full length (WT), mutant and deletion cDNA constructs of S100A11 were inserted into the pDNR-1r (CMV-CMV) vector to express the constructs as N-terminal enhanced green fluorescent protein (EGFP) fusion proteins. Immunoblot analysis, immunocytochemistry and immunoprecipitation Proteins were separated by SDS–polyacrylamide gel electrophoresis and transferred to nitrocellulose membranes. Primary antibodies raised against human S100A11 (1:1,000 dilution) (ProteinTech Group), Annexin A1 (1:1,000 dilution) (Abcam), Annexin A2 (1:1,000 dilution) (BD Transduction Laboratories), heat-shock cognate 70 kDa protein (1:6,000 dilution) (Hsc70; N69, kindly provided by Boris Margulis, Russian Academy of Sciences, St Petersburg, Russia), α-tubulin (1:5,000) (Abcam) and ErbB2 (1:1,000) (Fischer Thermo Scientific, MA) were used. This was followed by appropriate peroxidase-conjugated secondary antibodies (DAKO). Immunocytochemistry: cells on coverslips were fixed in paraformaldehyde and stained with indicated primary antibodies (1:300 dilution) including S100A11 and β-actin (Sigma). Samples were incubated with the appropriate Alexa Fluor-488- and Alexa Fluor-546/594-coupled secondary antibodies (1:1,000 dilution) (Molecular Probes) and images taken by confocal microscopy. IP was performed on lysates from HeLa or MCF7-ErbB2 cells overexpressing ANXA2-RFP and S100A11-GFP (WT or mutants) or only S100A11-turboGFP. Immunocomplexes were captured with RFP-Trap agarose beads (Chromotek) or turbo-GFP antibody (OriGene) coupled to sepharose-G beads and washed four times before immunoblot analysis (extended blots showing co-IP are presented in Supplementary Fig. 4 ). RNA extraction and quantitative PCR Total RNA was isolated using the NucleoSpin Total RNA Isolation Kit (Macherey-Nagel, Germany) and complementary DNA was synthesized using the TaqMan Reverse Transcription Kit (Roche) according to the manufacturers’ protocols. The primers used for quantitative PCR are listed in Supplementary Table 2 . Membrane integrity and cytometry Analysis of LAMP1 membrane levels: cells were incubated with anti-LAMP1 (Santa Cruz Biotechnology) antibody on ice for 30 min, fixed by paraformaldehyde and stained with Alexa Fluor-488 antibody. Plasma membrane integrity±scrape injury was performed by incubating cells (after injury) with impermeant 7-aminoactinomycin D (7-AAD) for 10 min followed by flow cytometry with a FACS (Becton Dickinson, CELLQUEST software). To measure membrane integrity, cells seeded in chamber slides were incubated with impermeant Hoechst-33342 in imaging media (Hank’s balanced salt solution with 10 mM HEPES and 1% FCS, pH 7.4) ±2 mM Ca 2+ . Hoechst-33342 uptake was imaged by a Carl Zeiss Axiovert 200M fluorescence time-lapse microscope and analysed using MetaMorph software. Cell death by PI exclusion assay was measured with an image-based Celigo cytometer (Brooks) according to manufacturer’s instructions. Membrane-wounding experiments These experiments were performed as detailed elsewhere [34] , [35] and described here briefly. Glass bead injury: cells were injured by rolling glass beads (425–600 μm, acid washed; Sigma) in cell-imaging media (CIM—Hank’s balanced salt solution+10 mM Hepes+2 mMCa 2+ , pH 7.4) containing 2 mg ml −1 lysine-fixable 10-kDa FITC-dextran. After healing at 37 °C for 5 min, cells were transferred to CIM containing 2 mg ml −1 lysine-fixable 10-kDa tetramethyl rhodamine isothicyanate (TRITC)-dextran for another 5 min. After paraformaldehyde fixation, the number of FITC-positive (total wounded cells) and TRITC-positive cells (wounded cells that have not resealed) were counted. Laser injury: cells were injured in CIM with 1 μg μl −1 of FM1-43 dye by selecting a small region (1–5 μm 2 ) and irradiating with a pulsed laser (AblateTM). Cells were imaged every 10 s starting before injury and continuing for 3–5 min following injury. For no repair control, cells were injured in Ca 2+ -free PBS containing 1 μg μl −1 of FM dye. The hardware was controlled using Slidebook 5.0 (Intelligent Imaging Innovations Inc., Denver) and the same software was used to measure the kinetics of repair by monitoring cellular FM dye fluorescence as change in intensity (Δ F / F 0) during the course of imaging. 3D matrigel invasion assay Cells were incubated overnight to form spontaneous spheroids on an inverted lid in a hanging drop containing 2.5 × 10 5 cells in RPMI tissue culture media (TCM) (GIBCO) with 10% FCS (GIBCO). The day after the spheroids were transferred to a layer of polymerized Matrigel (growth factor reduced; Becton Dickenson) diluted 1:1 with TCM. The spheroids were covered with a sealing layer of Matrigel mix and the TCM was added to cover the cells. The extent of the outgrowth was carefully followed up to 4 days. Images were taken with Olympus 1X71 light microscope supplemented with Cella P software. How to cite this article: Jaiswal, J. K. et al. S100A11 is required for efficient plasma membrane repair and survival of invasive cancer cells. Nat. Commun. 5:3795 doi: 10.1038/ncomms4795 (2014).